CHOLINE TRANSPORTER-LIKE1 is required for sieve plate development to mediate long-distance cell-to-cell communication Phloem, a plant tissue responsible for long-distance molecular transport, harbours specific junctions, sieve areas, between the conducting cells. To date, little is known about the molecular framework related to the biogenesis of these sieve areas. Here we identify mutations at the CHER1/AtCTL1 locus of Arabidopsis thaliana . The mutations cause several phenotypic abnormalities, including reduced pore density and altered pore structure in the sieve areas associated with impaired phloem function. CHER1 encodes a member of a poorly characterized choline transporter-like protein family in plants and animals. We show that CHER1 facilitates choline transport, localizes to the trans-Golgi network, and during cytokinesis is associated with the phragmoplast. Consistent with its function in the elaboration of the sieve areas, CHER1 has a sustained, polar localization in the forming sieve plates. Our results indicate that the regulation of choline levels is crucial for phloem development and conductivity in plants. Multicellular organisms have diverse cellular structures to facilitate cell communication, such as receptors, channels and junction structures. Choline metabolism and transport has been known for a long time as a major factor for cell communication in animals. Choline is classified as an essential nutrient for humans and serves as a precursor for the synthesis of both signalling and major membrane phospholipids, as well as (glycine) betaine and the neurotransmitter acetylcholine. Interference with choline uptake, transport or metabolism has been implicated in severe developmental defects and neurological disorders like Alzheimer and Parkinson’s [1] . Inter- and intracellular choline transport are mediated by different transporter systems such as the polyspecific organic cation transporters, the high-affinity choline transporters (CHTs) and the intermediate-affinity choline transporter-like proteins (CTLs) [2] , [3] . CHT1 is almost exclusively expressed in cholinergic neurons and is required for the reuptake of choline from the synaptic cleft into presynaptic neurons [4] , [5] , [6] , [7] , whereas the ubiquitous expression of CTL1/SLC44A1 in mammalian tissues suggest that choline transport is also required for more general cellular functions like phospholipid biosynthesis [3] , [8] , [9] , [10] , [11] , [12] . Interestingly, it has recently been suggested that CTL4/SLC44A4 may have a specific role in the synthesis of non-neuronal acetylcholine [13] . Little is known about choline transport in plants. Early studies using isotope-labelled choline indicated that the compound can be transported by carriers into plant cells. Also phosphocholine, a compound derived from choline, is found in xylem exudate. This organic phosphate ester might serve for phosphate and nitrogen storage and is distributed by the vascular system throughout the plant [14] , [15] . The idea that choline can be taken up from the media and distributed within the plant is further supported by the observation that externally supplied choline can rescue the developmental defects of xipotl , a phosphocholine biosynthesis mutant [16] . Choline might also be transported by the proline transporter BvBet/ProT1, which is expressed in phloem and xylem parenchyma cells of sugar beet [17] . Furthermore, observations made in bean ( Phaseolus vulgaris ) and soybean ( Glycine max ) suggest that extracellular choline is important for plant–pathogen interactions [18] . The conducting tissues for long-distance transport in plants are xylem and phloem ( Fig. 1a ). Phloem is required for the distribution of photosynthetic products, hormones, RNA, peptides and other molecules from source to sink tissues. The phloem tissue consists of phloem parenchyma cells, sieve tube elements and companion cells (CCs). Transport occurs through sieve tube elements, narrow elongated cylindrical cells, adjusted to each other and forming a network spanning the entire length of the plant. The cell walls between connecting sieve elements (SEs), called sieve plates, are perforated by a large number of pores, enlarged plasmodesmata, which enable intercellular transport and communication ( Fig. 1b ). Three major components represent the simplified structure of plasmodesmata: a tube that establishes plasma membrane continuity between adjacent cells, a central axial element derived from endoplasmic reticulum (desmotubule) and the cell wall surrounding the plasma membrane [19] , [20] . The conductivity of the sieve tubes can be regulated via callose (β-1,3-glucan) deposition at the neck region of plasmodesmata in the sieve plates [21] . Callose has been shown to be involved in the regulation of the sieve pore diameter. In cals7 mutants reduced callose deposition at the sieve plate leads to a reduced number of open pores per sieve plate, smaller diameter sieve pores and impaired phloem transport [22] , [23] . But also over accumulation of callose, as shown by the phloem-specific expression of a gain of function mutant of CalS3, inhibits phloem conductivity [24] , suggesting that callose deposition at the sieve plate has to be tightly regulated. The only gene identified so far which is specifically required to establish phloem identity is altered phloem development (APL), a MYB coiled-coil-type transcription factor [25] . Despite its importance for plant growth, the mechanisms regulating phloem development and especially sieve plate formation is still poorly understood. 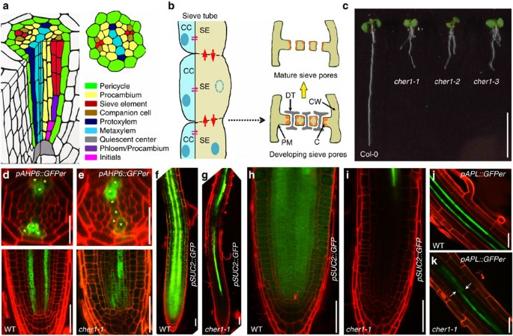Figure 1:cher1-1mutants show alteredpAHP6::GFPerexpression and abnormal phloem development. (a) Schematic presentation of theArabidopsisroot highlighting the vascular cylinder. (b) Schematic of sieve tube structure and sieve pore maturation. (c) Seedling phenotype of 6-day-old wild-type (Col-0),cher1-1,cher1-2andcher1-3. Scale bar, 1 cm. (d,e)pAHP6::GFPerin wild-type Col-0 (d) andcher1-1(e). Pericycle and protoxylem cells expressingpAHP6::GFPerare marked with yellow asterisks. Scale bars represent 50 μm for longitudinal and 25 μm for cross-sections. (f–i)pSUC2::GFPin wild-type Col-0 (f,h) andcher1-1(g,i) (the tip region is shown at higher magnification inhandi). (j,k)pAPL::GFPerin wild-type (j) andcher1-1(k). White arrows indicate the sites of fragmentedpAPL::GFPerexpression. Scale bar, 50 μm. Figure 1: cher1-1 mutants show altered pAHP6::GFPer expression and abnormal phloem development. ( a ) Schematic presentation of the Arabidopsis root highlighting the vascular cylinder. ( b ) Schematic of sieve tube structure and sieve pore maturation. ( c ) Seedling phenotype of 6-day-old wild-type (Col-0), cher1-1 , cher1-2 and cher1-3 . Scale bar, 1 cm. ( d , e ) pAHP6::GFPer in wild-type Col-0 ( d ) and cher1-1 ( e ). Pericycle and protoxylem cells expressing pAHP6::GFPer are marked with yellow asterisks. Scale bars represent 50 μm for longitudinal and 25 μm for cross-sections. ( f – i ) pSUC2::GFP in wild-type Col-0 ( f , h ) and cher1-1 ( g , i ) (the tip region is shown at higher magnification in h and i ). ( j , k ) pAPL::GFPer in wild-type ( j ) and cher1-1 ( k ). White arrows indicate the sites of fragmented pAPL::GFPer expression. Scale bar, 50 μm. Full size image In Arabidopsis , seven genes share sequence similarity to CTL genes in animals and yeast. Here, we show that one of the Arabidopsis CTL homologues, At3g15380 , named here as CHER1, mediates choline transport and loss-of-function results in an altered choline metabolite profile, defects in sieve plate and sieve pore formation and impaired phloem transport. CHER1 is expressed in several tissues, localizes to the trans-Golgi network (TGN) and transiently to the forming cell plate during cytokinesis. In addition, during early SE differentiation, CHER1 has a polar localization associated with the forming sieve plates. Together, our results indicate that a CTL-like protein functions in a choline transport process that is involved in sieve plate and sieve pore formation in plants. Isolation of cher1 mutants with altered AHP6 expression To identify novel regulators of vascular patterning and transport, we carried out a misexpression screen for pAHP6::GFPer , a cytokinin signalling inhibitor. pAHP6::GFPer is normally expressed in a highly specific pattern associated with xylem [26] ( Fig. 1d ), and its expression pattern is known to respond to the transport status of the phloem [27] . Screening ethyl methanesulfonate (EMS) mutagenized plants expressing pAHP6::GFPer resulted in the isolation of three mutants ( Fig. 1c ) with similar variable, often expanded pAHP6::GFPer expression (50%, n =20; Fig. 1e ), which we further characterized. An allelism test revealed that the three isolated mutants are allelic. cher1 mutants exhibit defects in root development All three cher1 mutant alleles are dwarf with defects in both shoot and root architecture ( Fig. 1c ). Shortly after germination, cher1 mutants develop a severe root growth phenotype that involves reduced primary root growth and lateral roots that grow approximately the same length as the primary root. Six–day-old cher1 seedlings develop a primary root about 10% of the length of a wild-type (WT) root ( Supplementary Fig. 1a ). Also the size of the root meristem region decreased during the first 5–6 dag as determined by propidium iodide-stained roots using confocal laser scanning microscope ( Supplementary Fig. 1b,c ). Severe swelling of ground tissue cells, abnormal root hair development and aberrant cell wall positioning are further characteristics of cher1-1 mutant ( Supplementary Fig. 1d,e ). Consistent with misexpression of pAHP6::GFPer, altered xylem specification was detected in the stele of cher1 mutants. Fuchsin staining of cher1 mutants revealed that the distinct patterning of meta- and protoxylem as observed in WT roots is abolished. The xylem in cher1-1 mutant is often discontinuous, some of the roots developed extra meta- or protoxylem files ( Supplementary Fig. 1f,g ). CHER1 is required for phloem patterning and conductivity To follow-up the pAHP6::GFPer misexpression aspect, which is informative for phloem function, we next analysed vascular conductivity in the cher1-1 mutant. In WT plants, green fluorescent protein (GFP) expressed under control of the CC-specific pSUC2 promoter ( pSUC2::GFP ) [28] is translocated from CC to SEs and unloaded symplastically into the root meristem ( Fig. 1f,h ). In cher1-1 mutant, the unloading of GFP from protophloem into the root meristem is blocked ( Fig. 1g,i ). Reduced symplastic movement was further observed in cher1-1 mutants expressing pSUC2::SpoGFP [29] , a Sporamin fused to GFP to increase the protein size ( Supplementary Fig. 1h–k ). These results indicate that the cher1-1 mutant is defective in symplastic transport through phloem. To understand the status of phloem conductivity, we next investigated phloem development in the cher1-1 mutants. Toluidine blue-stained cross-sections of 6-day-old cher1-1 roots revealed severe defects in procambium maintenance and phloem patterning. WT phloem poles consist of two CCs and two SEs ( Supplementary Fig. 1l ), whereas cher1-1 mutants exhibit an increased number of SE-like cells frequently extending into the procambial domain ( Supplementary Fig. 1m ). Furthermore, we observed a disrupted pattern of the phloem-specific pAPL::GFPer confirming that continuous phloem cell differentiation is unstable in cher1-1 mutant ( Fig. 1j,k ). CHER1 encodes a plant CHOLINE TRANSPORTER-LIKE protein To understand the role of the CHER1 gene product in regulating phloem morphogenesis or phloem conductivity, we next set out to better characterize the mutant locus. Rough mapping via a PCR-based positional cloning approach indicated the locus was between the markers J3-5079754 and J3-5255497 leaving a window of approximately 175 kb. Subsequent whole-genome re-sequencing (Illumina) revealed a premature STOP in the CHOLINE TRANSPORTER-LIKE (AtCTL1, At3g15380 ) [30] , [31] gene, which we rename here as CHER1 . Two other cher1 mutant alleles with premature STOP codons were identified from the same forward genetic screen. All three cher1 alleles ( cher1-1 (TGG→TAG at position 1403 of CDS) , cher1-2 (TGG→TGA at position 438 of CDS) and cher1-3 (CGA→TGA at position 946 of CDS)) and a T-DNA insertion mutant (SALK_065853; Fig. 2a ) segregate in a recessive manner. In addition, we were able to complement cher1-1 with a 3117-bp genomic DNA encompassing the CHER1 coding sequence and the 1,337 bp 5′-upstream region ( Fig. 2b ). The CHER1/At3g15380 locus encodes a protein of 700 amino acids, with ten predicted trans-membrane spanning domains (TMHMM Server v. 2.0) similar to the predictions of most CTL proteins from rat or human and other organisms [3] . In plants, seven genes including CHER1/At3g15380 have been annotated as potential CTL proteins in Arabidopsis based on their protein sequence similarity ( Supplementary Fig. 2a ). However, our in sillico analysis with the multiple alignment with CTL proteins from various organisms revealed that CHER1 is closest in homology to the animal CTL proteins and is distinct from the other six Arabidopsis CTL-like proteins ( Supplementary Fig. 2b,c ). 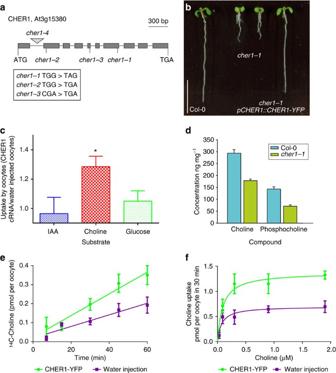Figure 2:CHER1facilitates choline transport. (a) Schematic view of the intron–exon structure ofCHER1and sites ofcher1-1,cher1-2,cher1-3mutations and T-DNA insertioncher1-4(SALK_065853). (b) Seedling phenotype of 6-day-old wild-type Col-0,cher1-1andcher1-1rescued withpCHER1::CHER1-YFP. Scale bar, 1 cm. (c) Choline, glucose and auxin (IAA) uptake byXenopusoocytes expressingCHER1cDNA. Auxin has been selected as a negative control and has been tested previously in oocytes69. Error bars=s.e.m. (n=6 independent experiments,P=0.0052 for 10 μM14C-choline by Student’st-test using GraphPad Prism 5). (d) Choline and phosphocholine levels in Col-0 andcher1-1roots. Error bars=s.d., three biological replicates were used forcher1-1and four biological replicates for wild type. (e) Time-dependent choline uptake at 0.3 μM14C-choline by CHER1-YFP-expressing and water-injected oocytes. After subtraction of the background, the linear regression indicated a twofold difference in the slope between water-injected and CHER1-YFP-injected oocytes. Representative of four separate experiments at low choline concentrations (0.3–1 μM), error bars represent the s.e.m. of four to six oocytes. (f) A kinetic analysis of choline transport shows that CHER1 expression increases theVmaxfrom 0.70 to 1.37 pmol/30 min without changing theKm(0.07 versus 0.09 μM). Good fits (R2=0.96 for CHER-YFP- and 0.88 for water-injected oocytes, 24 oocytes for each condition, nonlinear fitting was done using GraphPad Prism 5) were obtained with a simple Michaelis–Menten equation after subtraction of the baseline measured in the presence of 104M unlabelled choline. Representative of three separate experiments. Figure 2: CHER1 facilitates choline transport. ( a ) Schematic view of the intron–exon structure of CHER1 and sites of cher1-1 , cher1-2 , cher1-3 mutations and T-DNA insertion cher1-4 (SALK_065853). ( b ) Seedling phenotype of 6-day-old wild-type Col-0, cher1-1 and cher1-1 rescued with pCHER1::CHER1-YFP . Scale bar, 1 cm. ( c ) Choline, glucose and auxin (IAA) uptake by Xenopus oocytes expressing CHER1 cDNA. Auxin has been selected as a negative control and has been tested previously in oocytes [69] . Error bars=s.e.m. ( n =6 independent experiments, P =0.0052 for 10 μM 14 C-choline by Student’s t -test using GraphPad Prism 5). ( d ) Choline and phosphocholine levels in Col-0 and cher1-1 roots. Error bars=s.d., three biological replicates were used for cher1-1 and four biological replicates for wild type. ( e ) Time-dependent choline uptake at 0.3 μM 14 C-choline by CHER1-YFP-expressing and water-injected oocytes. After subtraction of the background, the linear regression indicated a twofold difference in the slope between water-injected and CHER1-YFP-injected oocytes. Representative of four separate experiments at low choline concentrations (0.3–1 μM), error bars represent the s.e.m. of four to six oocytes. ( f ) A kinetic analysis of choline transport shows that CHER1 expression increases the V max from 0.70 to 1.37 pmol/30 min without changing the K m (0.07 versus 0.09 μM). Good fits ( R 2 =0.96 for CHER-YFP- and 0.88 for water-injected oocytes, 24 oocytes for each condition, nonlinear fitting was done using GraphPad Prism 5) were obtained with a simple Michaelis–Menten equation after subtraction of the baseline measured in the presence of 10 4 M unlabelled choline. Representative of three separate experiments. Full size image CHER1 facilitates choline transport The first CTL protein was isolated by screening a cDNA library from the Torpedo lobe, which is highly enriched in neurons to identify genes able to suppress the growth defects of a yeast mutant lacking choline transport and reduced choline metabolism [9] , [32] . Choline uptake experiments performed with CTL1 and CTL2 from different organisms using various heterologous cell systems showed that these CTL proteins can facilitate choline transport across membranes [9] , [32] , [33] , [34] , [35] , [36] . To test whether CHER1 also has the capability to transport choline, uptake experiments were performed using Xenopus oocytes. Expression of CHER1-GFP fusion proteins in the oocytes revealed that the tagged protein localizes primarily to intracellular compartments. However, the high levels of exogenous protein produced in the oocytes allow a small portion to be localized in the plasma membrane because of cell membrane trafficking, and the expression of in vitro transcribed tagged CHER1 RNA was able to increase choline uptake 1.3-fold ( Fig. 2c ) in the oocytes, which is similar to the uptake rates observed with tagged human CTL1 ( Supplementary Fig. 3a ). Both endogenous and CHER1-related choline uptake were time ( Fig. 2e and Supplementary Fig. 3a ) and temperature ( Supplementary Fig. 3b ) dependent. The time-dependent uptake at 0.3 μM 14C-choline revealed a twofold difference in the slope between water-injected and CHER1-YFP-injected oocytes ( Fig. 2e ). Moreover, the transport kinetics analysis showed that CHER1 increased the Vmax of a high affinity component of choline transport in the oocytes ( Fig. 2f ). A similar effect on Vmax has been observed previously with rat rCTL1a and rCTL1b proteins [36] . We observed a stimulatory effect of low pH on choline uptake in the presence of CHER1 ( Supplementary Fig. 3c ). In contrast, the transport of indole-3-acetic acid (IAA) and glucose by oocytes was not affected by the expression of CHER1 ( Fig. 2c ). To determine whether the loss of function mutations in CHER1 cause a reduction in choline and phosphocholine levels, we measured the total content of these molecules in the root of 7-day-old seedlings. The quantification revealed a significant reduction of Cho (40%, P <0.0001 Student’s t -test) and PCho (51%, P <0.0001, Student’s t -test) content in cher1-1 compared with that present in WT plants ( Fig. 2d ), indicating that CHER1 may be involved in the regulation and/or maintenance of choline metabolite levels in plants. Furthermore, we analysed the expression of pAPL::GFPer and the distribution of the freely moving GFP driven by the phloem CC-specific pSUC2 promoter during phloem development in the biosynthetic xipotl mutant, which also shows reduced levels of choline and phosphocholine [16] , [37] . Similar to cher1-1 , we observed a reduced movement and unloading defects of pSUC2::GFP ( Supplementary Fig. 4a–d ), in addition to the fragmented expression pattern of pAPL::GFPer ( Supplementary Fig. 4e,f ) in xipotl phloem and an increased number of SE-like cells in the root cross-section ( Supplementary Fig. 4g,h ). Taken together, these data indicate that CHER1 facilitates choline transport and maintains choline homeostasis during root (and phloem) development in Arabidopsis . CHER1 localizes to the TGN, forming cell- and sieve-plates We next investigated the subcellular localization of CHER1 in the meristematic cells of Arabidopsis root by expressing a functional pCHER1::CHER1-YFP in WT and cher1-1 mutants. We found that pCHER1::CHER1-YFP displayed a punctate pattern in the cytosol in close vicinity to the Golgi marker CD3-967-RFP [38] and colocalizes with the TGN/EE (early endosome) labelled by VHA-a1-RFP ( Fig. 3a–c ). Transmission electron microscopy of immunogold labelled ultrathin cryosections using GFP antibodies confirmed the presence of pCHER1::CHER1-YFP in the TGN/EE ( Fig. 3d ). Notably, in the mitotic cells, pCHER1::CHER1-YFP is present at the sides of centrifugally extending cell plates as indicated by the ring-like localization in a three-dimensional (3D) projection ( Fig. 3e–h ; Supplementary Movie 1 ). This localization suggests that pCHER1::CHER1-YFP accumulates at the phragmoplast, the site where vesicles are transported to the expanding cell plate. 4',6-Diamidino-2-phenylindole staining of cortex and epidermis cells expressing pCHER1::CHER1-YFP shows a specific requirement for CHER1 at the cell plate during the telophase stage of cell division ( Fig. 3h ). 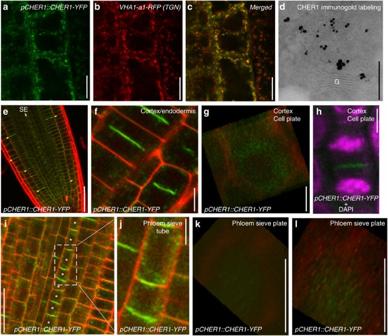Figure 3: CHER1 localizes to TGN, nascent cell plates and in phloem precursor cells to the sites of forming sieve plates. (a–c) Colocalization ofpCHER1::CHER1-YFPwith TGN markerVHA-a1-RFP.Scale bar, 7.5 μm. (d) Immunogold labelling of CHER1 inArabidopsisroot. G, Golgi. Scale bar, 250 nm. (e)pCHER1::CHER1-YFPexpression in phloem and outer layers of the root. Yellow arrows indicate cell plate-specificCHER1expression in outer layers of the root; white arrow indicates sieve element-specificCHER1expression. Scale bar, 50 μm. (f)pCHER1::CHER1-YFPexpression in cortex and epidermis cells. Scale bar, 7.5 μm. (g)pCHER1::CHER1-YFPring-like localization in a 3D projection at the cell plate of cortex and endodermis cells. Scale bar, 5 μm. (h) 4',6-Diamidino-2-phenylindole (DAPI) staining of endodermis cell expressingpCHER1::CHER1-YFP. Scale bar, 7.5 μm. (i,j) Polar CHER1 localization in the early phloem sieve elements. Protophloem sieve elements are marked with asterisks. Scale bar, 25 μm. (k,l) Sustained expression pattern ofCHER1in sieve plates in a 3D projection. Scale bars, 5 μm. Figure 3: CHER1 localizes to TGN, nascent cell plates and in phloem precursor cells to the sites of forming sieve plates. ( a – c ) Colocalization of pCHER1::CHER1-YFP with TGN marker VHA-a1-RFP. Scale bar, 7.5 μm. ( d ) Immunogold labelling of CHER1 in Arabidopsis root. G, Golgi. Scale bar, 250 nm. ( e ) pCHER1::CHER1-YFP expression in phloem and outer layers of the root. Yellow arrows indicate cell plate-specific CHER1 expression in outer layers of the root; white arrow indicates sieve element-specific CHER1 expression. Scale bar, 50 μm. ( f ) pCHER1::CHER1-YFP expression in cortex and epidermis cells. Scale bar, 7.5 μm. ( g ) pCHER1::CHER1-YFP ring-like localization in a 3D projection at the cell plate of cortex and endodermis cells. Scale bar, 5 μm. ( h ) 4',6-Diamidino-2-phenylindole (DAPI) staining of endodermis cell expressing pCHER1::CHER1-YFP . Scale bar, 7.5 μm. ( i , j ) Polar CHER1 localization in the early phloem sieve elements. Protophloem sieve elements are marked with asterisks. Scale bar, 25 μm. ( k , l ) Sustained expression pattern of CHER1 in sieve plates in a 3D projection. Scale bars, 5 μm. Full size image Whereas in most root meristem cells, pCHER1::CHER1-YFP is predominantly found at the TGN or at the phragmoplast in dividing cells, in SE cells pCHER1::CHER1-YFP exhibited a specific subcellular localization, in which CHER1-YFP accumulates in a polar manner at the central domain of the developing sieve plate ( Fig. 3e,i–l ). Compared with the transient ring-like localization in nascent cell plates ( Fig. 3g ), CHER1-YFP in the central domain of sieve plates is more sustained ( Fig. 3k,l ; Supplementary Movie 2 ). These data suggest that CHER1 has a specific function in the elaboration of the sieve plates/pores. Continuous vesicle trafficking maintains CHER1 polarity In (cholinergic) neurons, acetylcholine synthesis is maintained by the high-affinity CHT1, which transports choline across the plasma membrane. By influencing CHT1, endocytosis and trafficking choline uptake and hence acetylcholine biosynthesis can be regulated [39] . To investigate whether continuous membrane trafficking is required to maintain CHER1 polarity in SE cells, we treated seedlings expressing CHER1(cDNA)-YFP under control of an early phloem-specific promoter pEPM [40] with brefeldin A (BFA). BFA is a fungal toxin that inhibits vesicle transport and involves GDP-GTP exchange factors for small G proteins of the ARF class (ARF GEFs). In plants, BFA has been shown to block endocytic recycling of certain proteins and causes an aggregation of endosomes (including TGN) and internalized endocytic cargos into so-called BFA compartment [41] . In untreated seedlings, we observed pEPM::CHER1(cDNA)-YFP expression at the TGN and a polar pattern in phloem precursor cells ( Fig. 4a,b ). By contrast, BFA treatment caused rapid intracellular aggregation of CHER1 proteins into BFA compartments and loss of the polar pattern in the early sieve plates ( Fig. 4c,d ), indicating that continuous vesicle trafficking is required for creating CHER1 polarization in SE. Furthermore, we analysed the behaviour of two dynamin-related proteins, DRP1A and DRP1C, which are involved in the clathrin-mediated endocytosis in plants [42] , [43] , [44] . As previously reported, both DRP1A and DRP1C localize to the cell plate and the plasma membrane of expanding and fully expanded interphase cells [44] , [45] . Notably, we found that both DRP1A and DRP1C exhibit a similar polarized pattern to that of CHER1 in SE cells ( Fig. 4e–h ). Taken together, our observation here suggests that a BFA-sensitive endocytotic recycling mechanism might be involved in the maintenance of the polar CHER1 pattern in SE cells. 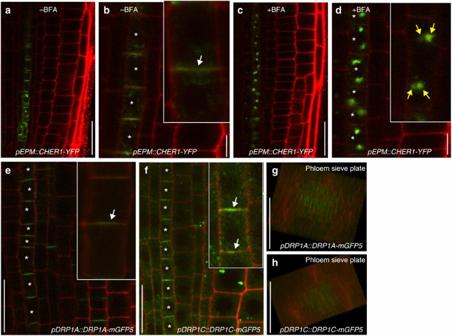Figure 4: Continuous vesicle trafficking is required for establishing CHER1 polarization and sustained pattern maintenance in the developing sieve plates. (a,b)pEPM::CHER1-YFPexpression in early sieve elements. Asterisks indicate phloem sieve elements and white arrows indicate polar CHER1 localization in the magnified image (b). Scale bars, 25 μm foraand 5 μm forb. (c,d)pEPM::CHER1-YFPexpression after 30 min of 50 μM BFA treatment. Asterisks indicate phloem sieve elements and yellow arrows indicate BFA compartments in the magnified image (d). Scale bars represent 25 μm (c) and 5 μm (d). (e)pDRP1A:DRP1A-mGFP5expression in the early sieve elements. (f)pDRP1C:DRP1C-mGFP5expression in the early sieve elements. Asterisks indicate phloem sieve elements and white arrows indicate polar DRP1A and DRP1C expression pattern. (g,h) Sustained expression pattern ofDRP1A(g) andDRP1C(h) in sieve plates in a 3D projection. Scale bars, 5 μm. Figure 4: Continuous vesicle trafficking is required for establishing CHER1 polarization and sustained pattern maintenance in the developing sieve plates. ( a , b ) pEPM::CHER1-YFP expression in early sieve elements. Asterisks indicate phloem sieve elements and white arrows indicate polar CHER1 localization in the magnified image ( b ). Scale bars, 25 μm for a and 5 μm for b . ( c , d ) pEPM::CHER1-YFP expression after 30 min of 50 μM BFA treatment. Asterisks indicate phloem sieve elements and yellow arrows indicate BFA compartments in the magnified image ( d ). Scale bars represent 25 μm ( c ) and 5 μm ( d ). ( e ) pDRP1A:DRP1A-mGFP5 expression in the early sieve elements. ( f ) pDRP1C:DRP1C-mGFP5 expression in the early sieve elements. Asterisks indicate phloem sieve elements and white arrows indicate polar DRP1A and DRP1C expression pattern. ( g , h ) Sustained expression pattern of DRP1A ( g ) and DRP1C ( h ) in sieve plates in a 3D projection. Scale bars, 5 μm. Full size image CHER1 is required for sieve plate and sieve pore elaboration The intriguing polar localization of CHER1 in SE cells suggests that CHER1 may have a role in the elaboration of sieve plates. Using serial block-face scanning electron microscopy (SBEM) [46] , we next compared serial sectioned roots of two WT (from 235 to 562 μm and from 210 to 525 μm from the root tip) and two cher1-1 (from 162 to 408 μm and from 129 to 445 μm from the root tip) seedling root tips from the quiescent center (QC) to the region in the root where enucleated SEs start to be formed ( Fig. 5a ). In addition, we analysed the sieve plates in mature cher1-1 and WT roots ( Fig. 6c,d ). The data revealed that, despite having a reduced sieve plate area (17.16 μm 2 in cher1-1 and 20.01 μm 2 in WT average), cher1-1 mutants have a reduced sieve pore density (1.86 pores per μm 2 in cher1-1 and 2.35 pores per μm 2 in WT average) when compared with WT ( Fig. 5b–d ). As sieve pores are necessary for the translocation of various micro- and macromolecules from one phloem cell to the next and thereby enable long-distance transport throughout the plant body, having a reduced sieve pore number in cher1-1 is likely to explain the impaired transport of GFP in the phloem observed with proSUC2::GFP mentioned above. 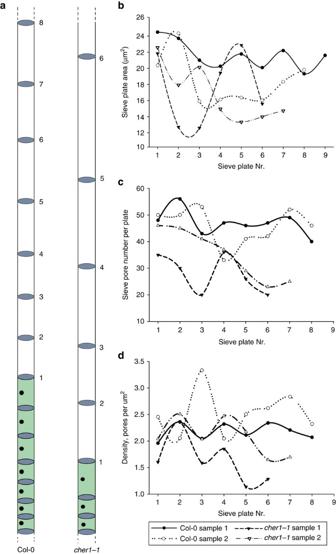Figure 5:Sieve pore density is reduced incher1mutant. (a) Schematic view of developing Col-0 andcher1-1sieve elements. Sieve elements incher1mutant become elongated earlier than in Col-0 roots. Sieve plates taken for analysis are numbered accordingly. (b–d) Analysis of sieve pore area (b), sieve pore number (c) and sieve pore density (d) in two independent wild-type Col-0 and twocher1-1roots. The plate between ‘green’ and ‘white’ cells is taken as a starting point for analysis. Figure 5: Sieve pore density is reduced in cher1 mutant. ( a ) Schematic view of developing Col-0 and cher1-1 sieve elements. Sieve elements in cher1 mutant become elongated earlier than in Col-0 roots. Sieve plates taken for analysis are numbered accordingly. ( b – d ) Analysis of sieve pore area ( b ), sieve pore number ( c ) and sieve pore density ( d ) in two independent wild-type Col-0 and two cher1-1 roots. The plate between ‘green’ and ‘white’ cells is taken as a starting point for analysis. 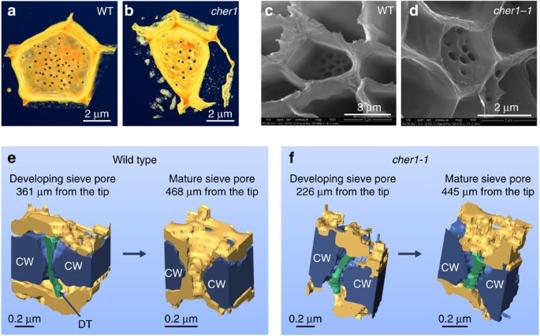Figure 6: CHER1 is required for sieve plate and sieve pore formation. (a,b) Reconstructed SBF-SEM images of wild-type Col-0 (at 377 μm;a) andcher1-1(at 310 μm;b) sieve plates. Scale bars, 2 μm. (c,d) SEM images of wild-type Col-0 (c) andcher1-1sieve plates (d). (e,f) Models of developing and mature sieve pores. The following sieve pores were selected to model 3D structure: developing and mature sieve pores in Col-0 (361 and 468 μm from the root tip correspondingly;e), developing and mature sieve pores incher1-1(226 and 445 μm from the root tip correspondingly;f). CW, cell wall; DT, desmotubule. Scale bars, 0.2 μm. Full size image Figure 6: CHER1 is required for sieve plate and sieve pore formation. ( a , b ) Reconstructed SBF-SEM images of wild-type Col-0 (at 377 μm; a ) and cher1-1 (at 310 μm; b ) sieve plates. Scale bars, 2 μm. ( c , d ) SEM images of wild-type Col-0 ( c ) and cher1-1 sieve plates ( d ). ( e , f ) Models of developing and mature sieve pores. The following sieve pores were selected to model 3D structure: developing and mature sieve pores in Col-0 (361 and 468 μm from the root tip correspondingly; e ), developing and mature sieve pores in cher1-1 (226 and 445 μm from the root tip correspondingly; f ). CW, cell wall; DT, desmotubule. Scale bars, 0.2 μm. Full size image As the SE differentiates, it undergoes a selective breakdown and all the remaining components become distributed along the wall [47] , [48] . Studies of SE formation in various plant species revealed that this process is accompanied by plasmodesmata enlargement and disintegration of the desmotubules, which leads to the formation of mature sieve plate pores [49] , [50] ( Fig. 1b ). Callose deposition around plasmodesmata has been suggested to have an important role in initiating this process [23] . Using the SBEM, we observed that during the differentiation of SEs the sieve pores are gradually losing the desmotubules, rigid structures derived from endoplasmic reticulum that run between two SEs. For our analysis, we selected the sieve plates at the junction between ‘grey’ (cell which still undergoes the selective breakdown) and ‘white’ (lacking most of cellular compartments) cells and additionally the sieve plates between already elongated and differentiated SEs ( Supplementary Fig. 5a ). We could not detect a significant difference in the sieve pore anatomy in the junction between ‘grey’ and ‘white’ cells in WT (361 μm from the root tip; left model in Fig. 6e and Supplementary Fig. 5b ,c) and the cher1-1 mutant (226 μm from the root tip; left model in Fig. 6f and Supplementary Fig. 5b ), where the sieve pores still retained the desmotubules. However, the analysis of the sieve pores in already developed SEs revealed a significant difference between WT and cher1-1 . The majority of sieve pores in the WT (468 μm from the root tip; right model in Fig. 6e and Supplementary Fig. 5b,c ) have lost the desmotubules, whereas cher1-1 sieve pores (445 μm from the root tip) still retained the desmotubules in the symplastic space (right model in Fig. 6f and Supplementary Fig. 5b,c ). Finally, we found that the sieve plate area, sieve pore number and sieve pore area are reduced in 30-day-old xipotl and cher1-1 roots compared with WT ( Supplementary Fig. 4i–k ). Taken together, our analyses indicate that the function of CHER1 as a facilitator of choline transport is required for the proper sieve pore formation in developing SEs. In fungi and animals, the shortage of notable ctl mutant phenotypes under non-stress/-induced conditions [9] , [51] , [52] has hampered so far the investigation of CTL-dependent developmental processes. Here we report the identification of CHER1 as a novel regulator of sieve plate formation and provide evidence that CHER1 is involved in maintaining choline homeostasis in the Arabidopsis root. Enucleated sieve tubes of the phloem form a conductive tissue to distribute various molecules within plants. In order to facilitate long-distance transport, the cell walls separating neighbouring sieve tubes are perforated by sieve pores. Despite its importance for growth and fitness of higher plants, little is known about the genetic regulation of phloem development. Both expression analysis of phloem marker genes and 3D-scanning electron microscopy (SEM) data revealed that our novel loss-of-function cher1 mutants fail to unload free (cytosolic) GFP from the phloem into the root tip and form a reduced number and structurally altered sieve pores in sieve plates. As phloem conductance is predicted to be directly linked to the density and size of pores on the sieve plate [53] , [54] , we propose that CHER1 is required for sieve plate elaboration and hence influences phloem long-distance transport and continuity. This is further supported by the initial observation that the expression domain of AHP6 , which is regulated by the function of phloem-derived phytohormone [27] , is expanded in cher1 mutants. Consistent with its role in phloem development, CHER1 accumulates at the sites of forming sieve plates but it is also localized to the TGN and forming cell plates in other root cell types. Endocytosis allows cells to adjust the protein composition and localization at the plasma membrane in response to developmental and environmental cues. This process has been shown to regulate the abundance and polarity of various transporters, such as CHT1 in human embryonic kidney and neuroblastoma cells [39] , [55] , [56] , [57] , [58] , aquaporins [59] and PIN-FORMED (PIN) auxin efflux carriers [60] , [61] , [62] in Arabidopsis . Our observation that CHER1 is rapidly endocytosed at forming cell plates suggests that a specific vesicle transport machinery is employed to continuously target CHER1 to the forming sieve plates. Consistent with data from transport assays performed with CTLs from various organisms [9] , [11] , [35] , expression of CHER1 in Xenopus oocytes increased choline uptake from the medium. As the loss of CHER1 results in reduced choline metabolite levels in the root, it is likely that CHER1-mediated maintenance of choline levels is crucial for proper root development. This notion is further supported by the phenotypic similarity of cher1 and the phosphocholine biosynthetic xipotl ( xpl) mutant [16] . At this stage, our work does not fully reveal the cellular process for which CHER1 is required for sieve plate development. Further investigations will be required to clarify the molecular and physiological function of CTLs in plants. For this analysis, the three cher1 alleles of Arabidopsis may provide an important resource. Plant materials and growth conditions WT Columbia (Col-0) mutants cher1-1 , cher1-2 and cher1–3 were isolated in a genetic screen based on EMS mutagenesis of the mobile phloem marker pAHP6::GFPer . The cher1-1 (Col-0) was crossed to Landsberg (Ler) to generate F2 mapping population. The information on mapping, sequencing and genotyping primers is provided in Supplementary Tables . cher1-4 (SALK_065853) was obtained from the Nottingham Arabidopsis Stock Centre. The reporter lines pAHP6::GFPer [26] , pAPL::GFPer [25] , pSUC2::GFP [28] , pSUC2- spoGFP [29] , VHA-a1–GFP [63] and pDRP1A:DRP1A-mGFP5 (ref. 45 ) have been described previously. Seedlings were grown vertically in Petri dishes on 1% agar, one-half of Murashige and Skoog (MS) basal salt mixture, 1% sucrose and 0.05% 4-morpholine ethanesulfonic acid (MES). Whole-genome re-sequencing Five microgram of purified genomic DNA in total volume of 50 and 700 μl nebulization buffer were added to a nebulizer. Shearing was performed for 6 min at 32–35 p.s.i. The recovered volume was 410 μl. The sample solution was purified and concentrated by column (Qiagen). End repair of the sheared fragments, addition of an A residue to the 3′ end of blunted fragments, and ligation of paired-end (PE) adaptors were according to the Illumina’s instructions. The entire adaptor-modified DNA was resolved on a 2% agarose gel (including 400 ng ml −1 ethidium bromide) run in 1 × TAE buffer (Bio-Rad) for 90 min at 120 V. Fragments of 300 b.p.s. were excised under illumination from a Dark Reader (Clare Chemical Research). The DNA was then isolated with a Gel Extraction Kit (Qiagen) and 1 μl (2.5 ng) was amplified by PCR for 12 cycles with the supplied Illumina PCR primers 1.1 and 1.2 (Illumina). PCR fragments were purified by PCR purification kit (Qiagen) and eluted with 50 μl elution buffer (Qiagen). The library yield was quantified by Nanodrop and diluted to 10 nM in EB buffer (Qiagen) supplemented with 0.1% Tween-20 for long-term storage at −20 °C. The DNA sample was sequenced by the Max Planck Institute for Developmental Biology, Tübingen, Germany, on an Illumina GAIIx instrument (Illumina). Whole-genome sequencing data were filtered and trimmed based on per based quality information using SHORE [30] . Quality controlled data were aligned against the A. thaliana reference sequence using GenomeMapper allowing for at most 10% of the read length to be involved in either gaps or mismatches [31] , [64] . Consensus calls were performed by SHORE consensus using default parameters. All confident mismatches within the 175-kb mapping interval were annotated according to their effect of gene integrity. The whole-genome sequencing data of cher1-1 have been deposited to the European Nucleotide Archive under accession code PRJEB6417. Transgenic work pAPL::GFPer , pAHP6::GFPer , pSUC2::GFP and pSUC2-spoGFP markers were introduced into cher1-1 mutant background by crossing and analyses were done on segregating F2 generations. Transgenic constructs were generated using the Multisite Gateway System (Invitrogen). A 3.1-kb genomic CHER1 fragment was amplified by PCR using primers 5′-AAAAAGCAGGCTATGAGAGGACCTTTAGGAGCAGTG-3′ (forward) and 5′-AGAAAGCTGGGTTGTGAGTAAGACTCTGAACCTCTTCC-3′ (reverse) and cloned into pDONR(Zeo) (Invitrogen) vector and verified by sequencing. Subsequently, the 1.3-kb sequence corresponding to the CHER1 promoter ( pCHER1 ) was amplified from Col-0 genomic DNA using primers 5′-ATAGAAAAGTTGCTACAAAACTAAGTCGTGCTCTGG-3′ (forward) and 5′-TTGTACAAACTTGACTTTGCCACAGCTATGTCTCTTCAC-3′ (reverse) and cloned into pDONRP4-P1R (Invitrogen). pCHER1 , CHER1 and YFP were combined into the multisite destination vector pBm43gw [65] and transformed by floral dipping [66] into Col-0 and cher1-1 mutant. To produce pEPM::CHER1(cDNA)-YFP , a 2.1-kb fragment was amplified from Col-0 cDNA by PCR using primers 5′-AAAAAGCAGGCTATGAGAGGACCTTTAGGAGCAGTG-3′ (forward) and 5′-AGAAAGCTGGGTTGTGAGTAAGACTCTGAACCTCTTCC-3′ (reverse), cloned into pDONR(Zeo) vector and verified by sequencing. pEPM [67] , CHER1 (cDNA) and YFP were combined into the multisite destination vector pBm43GW and transformed by floral dipping into Col-0. Anatomical analyses and confocal microscopy For serial sectioning, 5-day-old seedlings were incubated in a fixation solution (1 ml of 25% glutaraldehyde, 2.7 ml of 37% formaldehyde, 2.5 ml of NaPi and 18.8 ml of H2O) at 4 °C overnight. After the fixation, the plants were dehydrated in an ethanol gradient (10%, 30%, 50%, 70%, 96%, 2 × absolute ethanol), for at least 30 min at each step. Next, the seedlings were incubated in a 1:1 mix of absolute ethanol and solution A (100 ml of Basic resin, 1 g of Historesin activator (both from Leica Historesin embedding kit) and 2 ml of polyethylene glycol) overnight at room temperature. Consequently, the incubation solution was replaced with pure solution A and incubated for 2 h more at room temperature. For embedding, the roots were oriented horizontally next to each other in a plastic well. The well was next filled with a mix of solution A and Historesin hardener (15:1) and covered with a plastic and left for polymerization to take place. As many wells were produced separately, they were finally combined into one block and filled with the previously mentioned polymerization mix. Finally, the resin blocks with embedded roots were attached to the wooden blocks for sectioning. 3–5 μm sections were made on a Leica JUNG RM2055 microtome, using a Leica microtome knife (Leica disposable blades TC-65; Leica). Sections were stained in a 0.05% toluidine blue solution and visualized with a Leica 2500 Microscope (Leica). For fuchsin staining, seedlings were first cleared with acidified methanol (10 ml of methanol, 2 ml of concentrated HCl (37%) and 38 ml of H 2 O) and incubated at 55°–57 °C for 15 min. The acidified methanol was replaced with basic solution (7% NaOH in 60% ethanol) and incubated for 15 min at room temperature. The rehydration of the seedlings took place in several steps (40, 20 and 10% ethanol, 10 min each). The seedlings were stained for 5 min in 0.01% basic fuchsin solution, destained in 70% ethanol for 10 min and rehydrated again in the ethanol gradient (40, 20 and 10%). An equal amount of 50% glycerol was added to the 10% ethanol and the seedlings were incubated overnight. Finally, the seedlings were mounted in 50% glycerol on the glass slides. The images of various markers and fuchsin-stained roots were taken on Leica SP5 confocal microscope using a solid-state blue laser for GFP (480 nm/270 mW). CHER1, DRP1A and DRP1C localization were examined by confocal z-sectioning and 3D reconstruction. To inhibit the endosomal recycling, the roots were treated with 50 μM BFA (Invitrogen). Expression in Xenopus oocytes and choline uptake assays Xenopus laevis oocytes were prepared by excision and defolliculation using collagenase D (20 mg ml −1 , Roche Diagnostics), then injected with CHER1 RNA made with mMessage mMachine (Ambion) from the oocyte expression vector pOO2. Uptake measurements were performed after 3–4 days of incubation in Barth’s medium. Oocytes were incubated at room temperature with 14 C-choline (2.04 GBq mmol −1 , Perkin-Elmer) at 0.1–10 μM for the indicated times, then washed and solubilized for determination of the accumulated radioactivity. Immunogold labelling For immunogold labelling of ultrathin thawed cryosections, root tips were fixed with 4% (30 min) and 8% formaldehyde (2 h), embedded in gelatin and infiltrated with a mixture of polyvinylpyrrolidone and sucrose. Thawed ultrathin sections were labelled with rabbit anti-GFP antibodies (1:300; Abcam) and goat anti-rabbit IgG coupled to Nanogold (no. 2004; Nanoprobes). After silver enhancement (HQ Silver, 8 min; Nanoprobes), sections were embedded in methyl cellulose. SBEM SBEM is a method that is based on a combination of a microtome (3View, Gatan) mounted inside the SEM chamber and a sensitive back-scattered electron detector (Gatan) producing classic transmission electron microscopy-like images. The microtome repeatedly shaves resin-embedded specimen to form a fresh block face that is being imaged. After each cutting and imaging step, the specimen is moved up by desired Z-step, and the cycle is automatically repeated. The roots were fixed with 2.5% glutaraldehyde, 2% formaldehyde in 0.1 M Na-Cacodylate buffer (pH 7.4) supplemented with 2 mM CaCl 2 for 2–3 h at room temperature, and prepared using a previously described protocol [70] . Durcupan ACM resin (Fluka, Sigma-Aldrich) was mixed according to the manufacture’s recommendations. After standard dehydration steps, samples were embedded in silicone holders filled with 100% Durcupan and infiltrated for at least 2 h before polymerization at 60 °C. The roots were trimmed to the desired starting point from the tip using EM Ultracut UC6i ultramicrotome (Leica Mikrosysteme GmbH) and a diamond knife. The excess resin around the root was trimmed away and the specimen was mounted on a 3View pin. Finally, the sides of the specimen were covered with silver paint (Agar Scientific Ltd.) and the whole assembly was platinum-coated using Quorum Q150TS (Quorum Technologies, UK). Images were acquired with a FEG-SEM Quanta 250 (FEI), using a backscattered electron detector (Gatan) with 2.5-kV beam voltage, spot size 3 and pressure between 0.15 to 0.3 Torr. The block faces were cut with 40 nm increments. The images were first processed and segmented using Microscopy Image Browser, a self-developed programme written under Matlab environment, and further visualized in Amira (FEI Visualization Sciences Group). Scanning electron microscopy Arabidopsis tissue for SEM investigations of sieve plates was prepared as described previously [68] . In short, plants were shockfrozen in liquid nitrogen, freeze substituted in ethanol and the cytoplasm was digested in 0.5% Proteinase K and 8% Triton X-100 for 2 weeks. The tissue was washed, freeze dried, sputter coated and observed in a FEI Quanta 200 FEG SEM. How to cite this article: Dettmer, J. et al. CHOLINE TRANSPORTER-LIKE1 is required for sieve plate development to mediate long distance cell-to-cell communication. Nat. Commun. 5:4276 doi: 10.1038/ncomms5276 (2014).